Equivalence of wave–particle duality to entropic uncertainty Interferometers capture a basic mystery of quantum mechanics: a single particle can exhibit wave behaviour, yet that wave behaviour disappears when one tries to determine the particle’s path inside the interferometer. This idea has been formulated quantitatively as an inequality, for example, by Englert and Jaeger, Shimony and Vaidman, which upper bounds the sum of the interference visibility and the path distinguishability. Such wave–particle duality relations (WPDRs) are often thought to be conceptually inequivalent to Heisenberg’s uncertainty principle, although this has been debated. Here we show that WPDRs correspond precisely to a modern formulation of the uncertainty principle in terms of entropies, namely, the min- and max-entropies. This observation unifies two fundamental concepts in quantum mechanics. Furthermore, it leads to a robust framework for deriving novel WPDRs by applying entropic uncertainty relations to interferometric models. As an illustration, we derive a novel relation that captures the coherence in a quantum beam splitter. When Feynman discussed the two-path interferometer in his famous lectures [1] , he noted that quantum systems (quantons) display the behaviour of both waves and particles and that there is a sort of competition between seeing the wave behaviour versus the particle behaviour. That is, when the observer tries harder to figure out which path of the interferometer the quanton takes, the wave-like interference becomes less visible. This trade-off is commonly called wave–particle duality (WPD). Feynman further noted that this is ‘a phenomenon which is impossible... to explain in any classical way, and which has in it the heart of quantum mechanics. In reality, it contains the only mystery [of quantum mechanics].’ Many quantitative statements of this idea, so-called WPD relations (WPDRs), have been formulated [2] , [3] , [4] , [5] , [6] , [7] , [8] , [9] , [10] , [11] , [12] , [13] . Such relations typically consider the Mach–Zehnder interferometer (MZI) for single photons, see Fig. 1 . For example, a well-known formulation proven independently by Englert [2] and Jaeger et al . [3] quantifies the wave behaviour by fringe visibility, , and particle behaviour by the distinguishability of the photon’s path, . (See below for precise definitions; the idea is that ‘waves’ have a definite phase, while ‘particles’ have a definite location, hence and , respectively, quantify how definite the phase and location are inside the interferometer.) 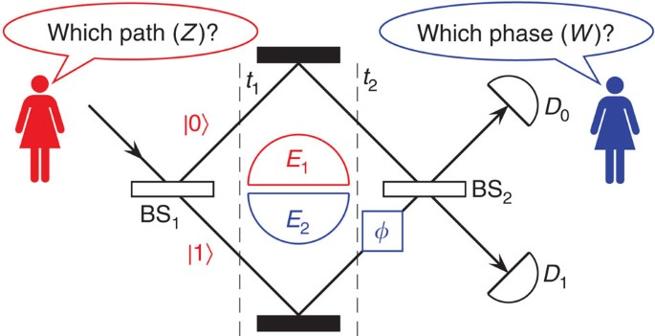Figure 1: MZI for single photons. Passing through the first beam splitter (BS) creates a superposition of which-path states, |0› and |1›, at timet1, then the system interacts with an environmentE=E1E2. Finally, at timet2, a phase shiftφis applied to the lower arm and the two beams are recombined on a second beam splitter. (While this is the typical setup, our framework also allowsEto play a more general role, for example, being correlated to the photon before it enters the MZI.) Our complementary guessing game proceeds as follows. In one game (coloured red), Alice tries to guess which of the two paths the photon took given that she has access to a portion ofEdenotedE1, which could be, for example, a gas of atoms whose internal states record information about the presence of a photon. In the other game (coloured blue), one of two phases,φ=φ0orφ=φ0+π, is randomly applied to the lower interferometer arm and Alice tries to guessφgiven that she has access to a different portion ofEdenotedE2, which could be, for example, the photon’s polarization. We argue that WPDRs impose fundamental trade-offs on Alice’s ability to win these two games. They found the trade-off: Figure 1: MZI for single photons. Passing through the first beam splitter (BS) creates a superposition of which-path states, |0› and |1›, at time t 1 , then the system interacts with an environment E = E 1 E 2 . Finally, at time t 2 , a phase shift φ is applied to the lower arm and the two beams are recombined on a second beam splitter. (While this is the typical setup, our framework also allows E to play a more general role, for example, being correlated to the photon before it enters the MZI.) Our complementary guessing game proceeds as follows. In one game (coloured red), Alice tries to guess which of the two paths the photon took given that she has access to a portion of E denoted E 1 , which could be, for example, a gas of atoms whose internal states record information about the presence of a photon. In the other game (coloured blue), one of two phases, φ = φ 0 or φ = φ 0 + π , is randomly applied to the lower interferometer arm and Alice tries to guess φ given that she has access to a different portion of E denoted E 2 , which could be, for example, the photon’s polarization. We argue that WPDRs impose fundamental trade-offs on Alice’s ability to win these two games. Full size image which implies when (full particle behaviour means no wave behaviour) and vice versa, and also treats the intermediate case of partial distinguishability. It has been debated, particularly around the mid-1990s [14] , [15] , [16] , whether the WPD principle, closely related to Bohr’s complementarity principle [17] , is equivalent to another fundamental quantum idea with no classical analogue: Heisenberg’s uncertainty principle [18] . The latter states that there are certain pairs of observables, such as position and momentum or two orthogonal components of spin angular momentum, which cannot simultaneously be known or jointly measured. Likewise, there are many quantitative statements of this idea, known as uncertainty relations (URs; see, for example, refs 19 , 20 , 21 , 22 , 23 , 24 , 25 , 26 , 27 , 28 , 29 ), and modern formulations typically use entropy instead of s.d. as the uncertainty measure, so-called entropic uncertainty relations (EURs) [24] . This is because the s.d. formulation suffers from trivial bounds when applied to finite-dimensional systems [21] , whereas the entropic formulation not only fixes this weakness but also implies the s.d. relation [22] and has relevance to information-processing tasks. At present, the debate regarding wave–particle duality and uncertainty remains unresolved, to our knowledge. Yet, Feynman’s quote seems to suggest a belief that quantum mechanics has but one mystery and not two separate ones. In this article, we confirm this belief by showing a quantitative connection between URs and WPDRs, demonstrating that URs and WPDRs capture the same underlying physics; see also refs 30 , 31 for some partial progress along these lines. This may come as a surprise, since Englert [2] originally argued that equation (1) ‘does not make use of Heisenberg’s uncertainty relation in any form’. To be fair, the UR that we show is equivalent to equation (1) was not known at the time of Englert’s paper, and was only recently discovered [25] , [26] , [27] , [28] , [29] . Specifically, we will consider EURs, where the particular entropies that are relevant to equation (1) are the so-called min- and max-entropies used in cryptography [32] . In what follows, we provide a general framework for deriving and discussing WPDRs—a framework that is ultimately based on the entropic uncertainty principle. We illustrate our framework by showing that several different WPDRs from the literature are in fact particular examples of EURs. Making this connection not only unifies two fundamental concepts in quantum mechanics, but also implies that novel WPDRs can be derived simply by applying already-proven EURs. Indeed, we use our framework to derive a novel WPDR for an exotic scenario involving a ‘quantum beam splitter’ [33] , [34] , [35] , [36] , where testing our WPDR would allow the experimenter to verify the beam splitter’s quantum coherence (see equation (17)). We emphasize that the framework provided by EURs is highly robust and entropies have well-characterized statistical meanings. Note that current approaches to deriving WPDRs often involve brute force calculation of the quantities one aims to bound; there is no general, elegant method currently in use. Our approach simply involves judicial application of the relevant UR. Moreover, we emphasize that URs can be applied to interferometers in two different ways. One involves preparation uncertainty, which says that a quantum state cannot be prepared having low uncertainty for two complementary observables, and it turns out that this is the principle relevant to the original presentation of equation (1) in ref. 2 . The other involves measurement uncertainty, which says that two complementary observables cannot be jointly measured [7] , [31] , and we discuss why this principle is actually what was tested in some recent interferometry experiments [34] , [37] . Framework We argue that a natural and powerful way to think of wave–particle duality is in terms of guessing games, and one’s ability to win such games is quantified by entropic quantities. Specifically, we consider complementary guessing games, where Alice is asked to guess one of two complementary observables—a modern paradigm for discussing the uncertainty principle. In the MZI, see Fig. 1 , this corresponds to either guessing which path the photon took or which phase was applied inside the interferometer. The which-path and which-phase observables are complementary and hence the uncertainty principle gives a fundamental restriction stating that Alice cannot be able to guess both observables. Our framework treats this complementary guessing game for binary interferometers. By binary, we mean any interferometer where there are only two interfering paths, that is, all other paths are classically distinguishable (from each other and from the two interfering paths). In addition to the MZI, this includes as special cases, for example, the Franson interferometer [38] (see Fig. 2 ) and the double-slit interferometer (see Fig. 3 ). Note that binary interferometers go beyond interferometers with two physical paths. For example, in the Franson interferometer, there are four possible paths but post-selecting on coincidence counts discards two of these paths, which are irrelevant to the interference anyway. 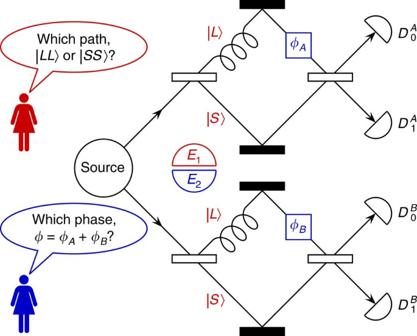Figure 2: Franson interferometer for entangled photons. In this interferometer, the ‘quanton’ consists of two photons. That is, a source produces time–energy entangled photons that each head separately towards a MZI that contains a long arm (depicted with extra loops) and a short arm. A simple model considers the 4D Hilbert space associated with the four possible paths: |SS›, |SL›, |LS› and |LL› withS=short path andL=long path. Two of these dimensions are post-selected away by considering only coincidence counts, that is, the photons arriving at the same time is inconsistent with the |SL› and |LS› paths. The remaining paths, |0›=|SS› and |1›=|LL›, are indistinguishable in the special case of perfect visibility and they produce interference fringes as one variesφ=φA+φB. Namely, the intensity of coincidence counts at detector pairoscillates withφ. Interaction with an environment system, or making the beam splitters asymmetric, may allow one to partially distinguish between |SS› and |LL›, and our entropic uncertainty framework can be applied to derive a trade-off, for example, of the form of equation (1). This trade-off captures the idea that Alice can either guess which path (|SS› versus |LL›) or which phase (φ=φ0versusφ=φ0+π), but she cannot do both (even if she extracts information from other systemsE1andE2). Figure 2: Franson interferometer for entangled photons. In this interferometer, the ‘quanton’ consists of two photons. That is, a source produces time–energy entangled photons that each head separately towards a MZI that contains a long arm (depicted with extra loops) and a short arm. A simple model considers the 4D Hilbert space associated with the four possible paths: | SS ›, | SL ›, | LS › and | LL › with S =short path and L =long path. Two of these dimensions are post-selected away by considering only coincidence counts, that is, the photons arriving at the same time is inconsistent with the | SL › and | LS › paths. The remaining paths, |0›=| SS › and |1›=| LL ›, are indistinguishable in the special case of perfect visibility and they produce interference fringes as one varies φ = φ A + φ B . Namely, the intensity of coincidence counts at detector pair oscillates with φ . Interaction with an environment system, or making the beam splitters asymmetric, may allow one to partially distinguish between | SS › and | LL ›, and our entropic uncertainty framework can be applied to derive a trade-off, for example, of the form of equation (1). This trade-off captures the idea that Alice can either guess which path (| SS › versus | LL ›) or which phase ( φ = φ 0 versus φ = φ 0 + π ), but she cannot do both (even if she extracts information from other systems E 1 and E 2 ). 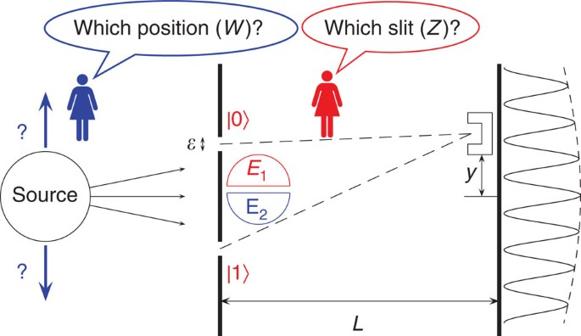Figure 3: Double-slit interferometer for arbitrary quantum particles. The first guessing game (coloured red) involves Alice guessing which slit the quanton goes through, given that she can measure a systemE1that has interacted with, and hence may contain information about, the quanton. In the second game (coloured blue), Bob randomly chooses the source’s vertical coordinate, and Alice tries to guess where the source was located, given some other systemE2and given where the quanton was finally detected. Note that the source’s location determines the relative phase between the which-slit states, |0› and |1›, and we assume that Bob chooses one of two possible locations such that the relative phase is either 0 orπ. Here, the state |0› (|1›) is defined as the pure state at the slit exit that one would obtain from blocking the bottom (top) slit. Our framework provides a WPDR that constrains Alice’s ability to win these complementary games. Furthermore, one can reinterpret the probability to win the second game, for the case whereE2is trivial, in terms of the traditional fringe visibility. The latter quantifies the amplitude of intensity oscillations as one varies the detector locationy. Note that varyingychanges the relative path lengths from the slits to the detector and hence is analogous to applying a relative phaseφbetween the two paths. (This assumes that the envelope function (dashed curve) associated with the interference pattern is flat over the range ofyvalues considered, which is often the case whenLis very large.) So, the double-slit fringe visibility is equivalent to the notion captured byin equation (7), where the detector is spatially fixed but a phase is varied, and we relateto our entropic measure of wave behaviour in the Methods section. Full size image Figure 3: Double-slit interferometer for arbitrary quantum particles. The first guessing game (coloured red) involves Alice guessing which slit the quanton goes through, given that she can measure a system E 1 that has interacted with, and hence may contain information about, the quanton. In the second game (coloured blue), Bob randomly chooses the source’s vertical coordinate, and Alice tries to guess where the source was located, given some other system E 2 and given where the quanton was finally detected. Note that the source’s location determines the relative phase between the which-slit states, |0› and |1›, and we assume that Bob chooses one of two possible locations such that the relative phase is either 0 or π . Here, the state |0› (|1›) is defined as the pure state at the slit exit that one would obtain from blocking the bottom (top) slit. Our framework provides a WPDR that constrains Alice’s ability to win these complementary games. Furthermore, one can reinterpret the probability to win the second game, for the case where E 2 is trivial, in terms of the traditional fringe visibility. The latter quantifies the amplitude of intensity oscillations as one varies the detector location y . Note that varying y changes the relative path lengths from the slits to the detector and hence is analogous to applying a relative phase φ between the two paths. (This assumes that the envelope function (dashed curve) associated with the interference pattern is flat over the range of y values considered, which is often the case when L is very large.) So, the double-slit fringe visibility is equivalent to the notion captured by in equation (7), where the detector is spatially fixed but a phase is varied, and we relate to our entropic measure of wave behaviour in the Methods section. Full size image Now we link wave and particle behaviour to knowledge of complementary observables. In the case of particle behaviour, the intuition is that particles have a well-defined spatial location, hence ‘particleness’ should be connected to knowledge of the path inside interferometer. For binary interferometers, there may be more than two physical paths, but only two of these are interfering. Hence, we only consider the two-dimensional (2D) subspace associated with the two which-path states of interest, denoted |0› and |1›. This subspace can be thought of as an effective qubit, denoted Q , and the standard basis of this qubit: corresponds precisely to the which-path observable. For example, in the double slit ( Fig. 3 ), |0› and |1› are the pure states that one would obtain at the slit exit from blocking the bottom and top slits, respectively. Wave behaviour is traditionally associated with having a large amplitude of intensity oscillations at the interferometer output. Indeed, this has been quantified by the so-called fringe visibility, see equation (7), but to apply the uncertainty principle we need to relate wave behaviour to an observable inside the interferometer. Classical waves (for example, water waves) are often modelled as having a well-defined phase and being spatially delocalized. The analogue in our context corresponds to the quanton being in a equally weighted superposition of which-path states. Hence, eigenstates of the ‘wave observable’ should live in the XY plane of the Bloch sphere, so we consider observables on qubit Q (the interfering subspace) of the form In terms of the guessing game, guessing the value of the wave (or which-phase) observable corresponds to guessing whether a phase of φ = φ 0 or φ = φ 0 + π was applied inside the interferometer (see, for example, Fig. 1 ). While φ 0 is a generic phase, its precise value will be singled out by the particular experimental setup. When the experimenter measures fringe visibility, this corresponds to varying φ 0 to find the largest intensity contrast, and mathematically we model this by minimizing the uncertainty within the XY plane, see the second of equations (4). Entropic view Our entropic view associates a kind of behaviour with the availability of a kind of information, or lack of behaviour with missing information, as follows: where H min and H max are the min- and max-entropies, defined below in equations (6), which are commonly used in quantum information theory, Z is the which-path observable in equation (2), W is the which-phase observable in equation (3) (whose uncertainty we optimize over the XY plane of the Bloch sphere) and E 1 and E 2 are some other quantum systems that contain information, and measuring these systems may help to reveal the behaviour (for example, E 1 could be a which-path detector and E 2 could be the quanton’s internal degree of freedom). Note that we use the same symbols ( Z , W and so on) for the observables as for the random variables they give rise to. Full behaviour (no behaviour) of some kind corresponds to the associated entropy in equations (4),  being zero (one). We formulate our general WPDR as This states that, for a binary interferometer, the sum of the ignorances about the particle and wave behaviours is lower bounded by 1 (that is, 1 bit). Equation (5) constrains Alice’s ability to win the complementary guessing game described above. If measuring E 1 allows her to guess the quanton’s path, that is, the min-entropy in the first of equations (4) is small, then, even if she measures E 2 , she still will not be able to guess the quanton’s phase, that is, the max-entropy in the second of equations (4) will be large (and vice versa). To be clear, equation (5) is explicitly an EUR, and it has been exploited to prove the security of quantum cryptography [39] . The usefulness of equation (5) for cryptography is due to the clear operational meanings of the min- and max-entropies [32] , which naturally express the monogamy of correlations as they give the distances to being uncorrelated ( H max ) and being perfectly correlated ( H min ). One can replace these entropies with the von Neumann entropy in equation (5) and the relation still holds; however, the min- and max-entropies give more refined statements about information processing since they are also applicable to finite numbers of experiments. From ref. 32 , the precise definitions of these entropies, for a generic classical-quantum state ρ XB , are where all logarithms are base 2 in this article. Here, p guess ( X | B ) denotes the probability for the experimenter to guess X correctly with the optimal strategy, that is, with the optimally helpful measurement on system B . Also, quantifies the secrecy of X from B , as measured by the fidelity F of ρ XB to a state that is completely uncorrelated. The fact that equation (5) can be thought of as a WPDR, and furthermore that it encompasses the majority of WPDRs found in the literature for binary interferometers, is our main result. To illustrate this, we consider the celebrated MZI, shown in Fig. 1 , since most literature WPDRs have been formulated for this interferometer. In the simplest case, one sends in a single photon towards a 50/50 (that is, symmetric) beam splitter, BS 1 , which results in the state , then a phase φ is applied to the lower arm giving the state . Finally, the two paths are recombined on a second 50/50 beam splitter BS 2 and the output modes are detected by detectors D 0 and D 1 . Fringe visibility is then defined as where is the probability for the photon to be detected at D 0 ; maximizes this probability over φ , whereas . In this trivial example, one has . However, many more complicated situations, for which the analysis is more interesting, have been considered in the extensive literature; we now illustrate how these situations fall under the umbrella of our framework with some examples. As a warm-up, we begin with the simplest known WPDR, the predictability–visibility trade-off. Predictability quantifies the prior knowledge, given the experimental setup, about which path the photon will take inside the interferometer. More precisely, where p guess ( Z ) is the probability of correctly guessing Z . Non-trivial predictability is typically obtained by choosing BS 1 to be asymmetric. In such situations, the following bound holds [4] , [5] : This particularly simple example is a special case of Robertson’s UR involving s.d. [30] , [31] , [40] , [41] . However, ref. 41 argues that equation (8) is inequivalent to a family of EURs where the same (Rényi) entropy is used for both uncertainty terms, hence one gets the impression that entropic uncertainty is different from wave–particle duality. On the other hand, ref. 41 did not consider the EUR involving the min- and max-entropies. For some probability distribution P ={ p j }, the unconditional min- and max-entropies are given by H min ( P )=−log max j p j and . We find that equation (8) is equivalent to which is an EUR proved in the seminal paper by Maassen and Uffink [23] , and corresponds to E 1 and E 2 in equation (5) being trivial. The entropies in equation (9) are evaluated for the state at any time while the photon is inside the interferometer. It is straightforward to see that and in Methods we prove that Plugging these relations into equation (9) gives equation (8). Let us move on to a more general and more interesting scenario where, in addition to prior which-path knowledge, one may obtain further knowledge during the experiment due to the interaction of the photon with some environment F , which may act as a which-way detector. Most generally, the interaction is given by a completely positive trace preserving map , with the input system being Q at time t 1 and output systems being Q and F at time t 2 , see Fig. 1 . The final state is , where the superscripts (1) and (2) indicate the states at times t 1 and t 2 . We do not require to have any special form to derive our WPDR, so our treatment is general. The path distinguishability is defined by , where p guess ( Z | F ) is the probability for correctly guessing the photon’s path Z at time t 2 given that the experimenter performs the optimally helpful measurement on F . We find that equation (1) is equivalent to where the entropy terms are evaluated for the state , which corresponds to E 1 = F and E 2 being trivial in equation (5). First, it is obvious from the operational meaning of the conditional min-entropy in the first of equations (6) that we have , and second we use our result equation (10) to rewrite equation (11) as equation (1). As emphasized in ref. 2 , we note that equation (1) and its entropic form equation (11) do not require BS 1 to be symmetric. Hence, accounts for both the prior Z knowledge associated with the asymmetry of BS 1 as well as the Z information gained from F . The above analysis shows that equations (1) and (8) correspond to applying the preparation UR at time t 2 (just before the photon reaches BS 2 ). Preparation uncertainty restricts one’s ability to predict the outcomes of future measurements of complementary observables. Thus, to experimentally measure or more generally , the experimenter removes BS 2 and sees how well he/she can guess which detector clicks, see Fig. 4a . Of course, to then measure , the experimenter reinserts BS 2 to close the interferometer. We emphasize that this procedure falls into the general framework of preparation uncertainty. 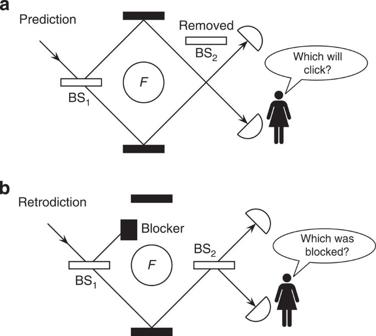Figure 4: Path prediction versus path retrodiction, in the MZI. (a) In the predictive scenario, the second beam splitter is removed and Alice tries to guess which detector will click. (b) In the retrodictive scenario, a blocker is randomly inserted into one of the interferometer arms and Alice tries to guess which arm was blocked (given the knowledge of which detector clicked). Figure 4: Path prediction versus path retrodiction, in the MZI. ( a ) In the predictive scenario, the second beam splitter is removed and Alice tries to guess which detector will click. ( b ) In the retrodictive scenario, a blocker is randomly inserted into one of the interferometer arms and Alice tries to guess which arm was blocked (given the knowledge of which detector clicked). Full size image On the other hand, URs can be applied in a conceptually different way. Instead of two complementary output measurements and a fixed input state, consider a fixed output measurement and two complementary sets of input states. Namely, consider the input ensembles from equations (2) and (3), now labelled as Z i ={|0›,|1›} and W i ={| w ± ›}, where i stands for ‘input’, to indicate the physical scenario of a sender inputting states into a channel. Imagine this as a retrodictive guessing game, where Bob controls the input and Alice has control over both F and the detectors. Bob chooses one of the ensembles and flips a coin to determine which state from the ensemble he will send, and Alice’s goal is to guess Bob’s coin flip outcome. Assuming BS 1 is 50/50, the two Z i states are generated by Bob blocking the opposite arm of the interferometer, as in Fig. 4b , while the W i states are generated by applying a phase (either φ 0 or φ 0 + π ) to the lower arm. It may not be common knowledge that this scenario leads to a different class of WPDRs, therefore we illustrate the difference in Fig. 4 . For clarity, we refer to introduced above as output distinguishability, whereas in the present scenario we use the symbol and call this quantity input distinguishability, defined by where is Alice’s probability to correctly guess Bob’s Z i state given that she has access to F and she knows that detector D 0 clicked at the output. Likewise, we define the notion of input visibility via: which quantifies how well Alice can determine W i given that she knows D 0 clicked. Now the uncertainty principle says there is a trade-off: if Alice can guess the Z i states well, then she cannot guess the W i states well and vice versa. In other words, Alice’s measurement apparatus, the apparatus to the right of the dashed line labelled t 1 in Fig. 1 , cannot jointly measure Bob’s Z and W observables. EURs involving von Neumann entropy have previously been applied to the joint measurement scenario [27] , [42] , we do the same for the min- and max-entropies to obtain (see Methods for details) which can now be applied to a variety of situations. As an interesting application of equation (14), we consider the scenario proposed in ref. 33 and implemented in refs 34 , 35 , 36 , where the photon’s polarization P acts as a control system to determine whether or not BS 2 appears in the photon’s path and hence whether the interferometer is open or closed, see Fig. 5 . Since P can be prepared in an arbitrary input state , such as a superposition, this effectively means that BS 2 is a ‘quantum beam splitter’, that is, it can be in a quantum superposition of being absent or present. The interaction coupling P to Q is modelled as a controlled unitary as in Fig. 5 . 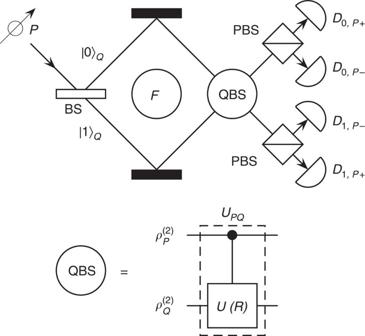Figure 5: Quantum beam splitter in the MZI. In this scenario, the second beam splitter is in a superposition of ‘absent’ and ‘present’, as determined by the polarization stateat timet2. The quantum beam splitter (QBS) can be modelled as a controlled unitary,UPQ=|H›‹H|P⊗Q+|V›‹V|P⊗U(R), whereU(R) is the unitary onQassociated with an asymmetric beam splitter with reflection probabilityR. Polarization-resolving detectors (PBS=polarizing beam splitter) on the output modes help to reveal the ‘quantumness’ of the QBS. In this case, the two visibilities are equivalent (see Methods) Figure 5: Quantum beam splitter in the MZI. In this scenario, the second beam splitter is in a superposition of ‘absent’ and ‘present’, as determined by the polarization state at time t 2 . The quantum beam splitter (QBS) can be modelled as a controlled unitary, U PQ =| H ›‹ H | P ⊗ Q +| V ›‹ V | P ⊗ U ( R ), where U ( R ) is the unitary on Q associated with an asymmetric beam splitter with reflection probability R . Polarization-resolving detectors (PBS=polarizing beam splitter) on the output modes help to reveal the ‘quantumness’ of the QBS. Full size image where we assume the dynamics are path preserving, that is, and , where is the reduced channel on Q , which implies that , that is, off-diagonal elements get scaled by a complex number κ with | κ |≤1. In equation (15), is evaluated for any pure state input from the XY plane of the Bloch sphere (for example, |+›). Now we apply equation (14) to this scenario and use equation (15) to obtain: which extends a recent result in ref. 13 to the case where F is non-trivial. This general treatment includes the special case where , corresponding to a closed interferometer with an asymmetric BS 2 . Ref. 37 [37] experimentally tested this special case. However, ref. 37 did not remark that their experiment actually tested a relation different from equation (1), namely, they tested a special case of equation (16). Similarly, ref. 34 tested equation (16) rather than equation (1), but they allowed to be in a superposition. At first sight, this seems to test the WPDR in the case of a quantum beam splitter (QBS), but it turns out that neither the visibility nor the distinguishability depends on the phase coherence in and hence the data could be simulated by a classical mixture of BS 2 being absent or present. Nevertheless, our framework provides a WPDR that captures the coherence in , by conditioning on the polarization P at the interferometer output (see Methods). For example, defining the polarization-enhanced distinguishability, , which corresponds to choosing E 1 = FP , we obtain the novel WPDR: which captures the beam splitter’s coherence (see Supplementary Note 4 for elaboration) and could be tested with the set-up in ref. 34 . The above examples use the environment solely to enhance the particle behaviour. To give a corresponding example for wave behaviour, that is, where system E 2 in equation (5) is non-trivial, the main result in ref. 11 is a WPDR for the case when the environment F is measured (after it has interacted with the quanton) and the resulting information is used to enhance the fringe visibility. This scenario is called quantum erasure, since the goal is to erase the which-path information stored in the environment to recover full visibility. This falls under our framework by taking E 2 to be the classical output of the measurement on the environment. For elaboration, see Supplementary Note 3 , where we also cast the main results of ref. 10 ( Supplementary Note 2 ) and ref. 12 ( Supplementary Note 3 ) within our framework. In summary, we have unified the wave–particle duality principle and the entropic uncertainty principle, showing that WPDRs are EURs in disguise. We leave it for future work to extend this connection to multiple interference pathways [6] . The framework presented here can be applied universally to binary interferometers. Our framework makes it clear how to formulate novel WPDRs by simply applying known EURs to novel interferometer models, and these new WPDRs will likely inspire new interferometry experiments. We note that all of our relations also hold if one replaces both min- and max-entropies with the well-known von Neumann entropy. Alternatively, one can use smooth entropies [29] , [39] , and the resulting smooth WPDRs may find application in the security analysis of interferometric quantum key distribution [43] , which often exploits the Franson set-up ( Fig. 2 ). Outline We emphasize that our treatment, in what follows, will be for a generic binary interferometer. We will first discuss our general treatment, then we will specialize to the predictive and retrodictive scenarios (see Fig. 4 ). Origin of general WPDR It is known that the min- and max-entropies satisfy the UR [29] : for any tripartite state where A is a qubit and Z and W are mutually unbiased bases on A . Noting that the which-path and which-path observables in equations (2) and (3) are mutually unbiased (for all φ 0 in equation (3), that is, for all W in the XY plane) gives our general WPDR in equation (5). Complementary guessing game The operational interpretation of equation (5) in terms of the complementary guessing game described, for example, in Figs 1 , 2 , 3 can be seen clearly as follows. While the min-entropy is related to the guessing probability via the first of equations (6), we establish a similar relation for the max-entropy. First, we prove (see Supplementary Note 1 ) that for a general classical-quantum state where X is binary, where the 1-norm is . Next we show (in Supplementary Note 1 ), for any positive semi-definite operators M and N , Combining equation 20 [20] with equation (19), and using the well-known formula , gives Now one can define generic measures of particle and wave behaviour directly in terms of the guessing probabilities: for some arbitrary quantum systems E 1 and E 2 , and rearrange equation (5) into the traditional form for WPDRs: This operationally motivated relation, which follows directly from equation (5), clearly imposes a restriction on Alice’s ability to win the complementary guessing game, since and are defined in terms of the winning probabilities. Below we show that becomes the fringe visibility when E 2 is discarded. Predictive WPDRs We now elaborate on our framework for deriving predictive WPDRs. Let us denote the quanton’s spatial degree of freedom as S , which includes the previously mentioned Q as a subspace. At time t 2 (see, for example, Fig. 1 )—the time just before a phase φ is applied and the interferometer is closed— S and its environment E are in some state , where again E = E 1 E 2 is a generic bipartite system. The preparation is arbitrary, that is, we need not specify what happened at earlier times, such as what the system’s state was at time t 1 (before the interaction between S and E ). While in general a binary interferometer may have more than two paths, all but two of these are non-interfering (by definition), hence we only consider the 2D subspace associated with the two which-path states of interest, denoted |0› and |1›. This subspace, defined by the projector Π=|0›‹0|+|1›‹1|, can be thought of as an effective qubit system Q . (Note that Q = S in the MZI.) Without loss of generality, we project the state onto this subspace and denote the resulting (renormalized) state as Experimentally, this corresponds to post-selecting on the interfering portion of the data. To derive predictive WPDRs, we apply equation (5) to the state in equation (25), where we associate the subsystems E 1 and E 2 of E with the particle and wave terms, respectively. For example, this approach gives the WPDRs discussed in ref. 2 , equations (1) and (8). To show this, we must prove equation (10), which relates our entropic measure of wave behaviour in the second of equations (4) to fringe visibility, and we now do this for generic binary interferometers. We remark that one can take equation (7) as a generic definition for fringe visibility, where the label D 0 is arbitrary, that is, it corresponds to some arbitrary detector. For generic binary interferometers, there is a phase shift φ applied just after time t 2 , as depicted in Fig. 1 . Let U φ =|0›‹0|+ e iφ |1›‹1| denote the unitary associated with this phase shift, and note that we only need to specify the action of U φ on the Q subspace since the state lives in this subspace. Finally, the quanton is detected somewhere, that is, system S is measured and a detector D 0 clicks. This measurement is a positive operator-valued measure (POVM) C ={ C 0 , C 1 ,…} on the larger space, system S rather than the subspace Q (for example, think of the double-slit case, where the detection screen performs a position measurement on S ). We associate the POVM element C 0 with the event of detector D 0 clicking. To prove equation (10), we need to restrict the form of C 0 . We show that equation (10) holds so long as C 0 is unbiased with respect to the which-path basis Z on the subspace Q . Fortunately, this condition is satisfied for all three types of interferometers in Figs 1 , 2 and 3 . More precisely, it is satisfied for the MZI provided BS 2 is 50/50, for the Franson case provided both BS 2 (the second beam splitters in Fig. 2 ) are 50/50 and for the double slit for some limiting choice of experimental parameters such as large L in Fig. 3 . We now state a general lemma that applies to all of these interferometers. Lemma 1 : Consider a binary interferometer where denotes the projection of POVM element C 0 onto the interfering subspace ( Q ). Suppose is proportional to a projector projecting onto a state from the XY plane of the Bloch sphere of Q , that is, for some 0< q ≤1, where | w + › is given by equation (3) for some arbitrary phase φ 0 , then it follows that where is given by equation (7) and H max ( W ) is evaluated for the state . Proof : In what follows, it should be understood that probabilities and expectation values are evaluated for the state . Suppose that is optimal in the sense that where , then we have where we denote Pauli operators by σ W =| w + ›‹ w + |−| w − ›‹ w − | and . The probability for D 0 to click is and maximizing this over φ gives Now, due to the geometry of the Bloch sphere, we have . Thus, and . This gives , completing the proof. Retrodictive WPDRs While we saw that the predictive approach allowed for any preparation but required complementary output measurements, the opposite is true in the retrodictive case, that is, the form of the output measurement is arbitrary while we require complementary preparations. The input ensembles Z i ={|0›, |1›} and W i ={| w + ›, | w − ›} can be generated by performing the relevant measurements on a reference qubit Q ′ that is initially entangled to the quanton S . Associating state ensembles with measurements on a reference system is a useful trick, for example, for deriving equation (14). Thus, at time t 1 (just after the quanton enters the interferometer; see Fig. 1 ) we introduce a qubit Q ′ that is maximally entangled to the interfering subspace ( Q ) of S , denoted by the state with . The dynamics after time t 1 is modelled as a quantum operation , defined in ref. 44 as a completely positive, trace non-increasing map that maps S → E 1 E 2 . The output of does not contain S because the quanton is eventually detected by a detector, at which point we no longer need a quantum description of the quanton’s spatial degree of freedom; we only care where it was detected. The map corresponds to a particular detection event; for concreteness say that detector D 0 clicking is the associated event. The probability for this event is the trace of the state after the action of , and renormalizing gives the final state Our framework applies the UR equation (5) to the state to derive retrodictive WPDRs. For example, this covers the scenario from the Discussion where involves two sequential steps. First, S interacts with an environment F inside the interferometer between times t 1 and t 2 , which corresponds to a channel mapping S to SF . Second, the quanton is detected at the interferometer output, say at detector D 0 , modelled as a map (·)=Tr S [ C 0 (·)] acting on S , where C 0 is the POVM element associated with detector D 0 clicking. Hence, we choose . Applying equation (5) to this case while choosing E 1 = F and E 2 to be trivial gives where the subscript means evaluating on the state in equation (31). Note that measuring Z on system Q ′ corresponds to sending the states {|0›, |1›} with equal probability through the interferometer, and similarly for W (with an inconsequential complication of taking the transpose of the W basis states). Realizing this, the first and second terms in equation (32) map onto and , respectively: Hence, equation (32) becomes equation (14). It remains to show that appearing in equation (14) can be replaced by for many cases of interest, such as the QBS case. We do this in the following lemma, where the proof is given in Supplementary Note 2 and is similar to the proof of Lemma 1. Lemma 2: Consider any binary interferometer with an unbiased input, that is, where the state at time t 1 is unbiased with respect to the which-path basis (of the form ). Let be the channel describing the quanton’s interaction with F inside the interferometer and let be the map that projects onto the subspace Π. Suppose is path preserving, that is, and and furthermore suppose commutes with , then where H max ( W ) is evaluated for the state . QBS example Finally, we treat the QBS shown in Fig. 5 . (Note that S = Q in the MZI.) This set-up involves first a quantum channel that describes the interaction of S with an environment F between times t 1 and t 2 , followed by another channel associated with the QBS that allows interaction of S with the polarization P , followed by a post-selected detection at D 0 . Together, these three steps form a quantum operation that maps S → FP , and hence this falls under our retrodictive framework. To prove equation (17), we apply equation (5) to the state in equation (31) while choosing E 1 = FP and E 2 to be trivial, giving We then use relations analogous to those in equations (33) and (34), where the former relation now involves conditioning also on the polarization P . Finally, we note that Lemma 2 applies to the QBS case. How to cite this article: Coles, P. J. et al . Equivalence of wave–particle duality to entropic uncertainty. Nat. Commun. 5:5814 doi: 10.1038/ncomms6814 (2014).